Brillouin light scattering from surface acoustic waves in a subwavelength-diameter optical fibre Brillouin scattering in optical fibres is a fundamental interaction between light and sound with important implications ranging from optical sensors to slow and fast light. In usual optical fibres, light both excites and feels shear and longitudinal bulk elastic waves, giving rise to forward-guided acoustic wave Brillouin scattering and backward-stimulated Brillouin scattering. In a subwavelength-diameter optical fibre, the situation changes dramatically, as we here report with the first experimental observation of Brillouin light scattering from surface acoustic waves. These Rayleigh-type surface waves travel the wire surface at a specific velocity of 3,400 m s −1 and backscatter the light with a Doppler shift of about 6 GHz. As these acoustic resonances are sensitive to surface defects or features, surface acoustic wave Brillouin scattering opens new opportunities for various sensing applications, but also in other domains such as microwave photonics and nonlinear plasmonics. The complex and intriguing dynamics of light and sound interactions in tiny optical waveguides have recently witnessed a renewed interest because of their experimental realization in emerging key areas of modern physics [1] . For instance, the micro and nanostructuring of photonic crystal fibres (PCFs) allows for a tight confinement of both photons and phonons, giving rise to new characteristics for Brillouin scattering fundamentally different from those of standard optical fibres. These include the generation of multiple high-frequency hybrid transverse and longitudinal acoustic waves (LAWs) trapped within the small core of microstructured optical fibres [2] , [3] , [4] , [5] . Strong photon–phonon coupling has also recently been reported in optical microcavities and new concepts have been introduced such as cavity or surface optomechanics [6] , [7] , [8] , Brillouin cooling [9] , on-chip Brillouin scattering [10] and microcavity lasers [10] , [11] , [12] . Moreover, the recent demonstration of simultaneous photonic and phononic bandgaps in nanostructured materials has led to the development of innovative opto-acoustic devices called phoxonic crystals [13] , [14] . In yet another example, tailorable Brillouin scattering was recently reported in nanoscale silicon waveguides [15] . Among other microdevices, photonic silica microwires are the tiny and as-yet underutilized cousins of optical fibres [16] , [17] . These hair-like slivers of silica glass, fabricated by tapering optical fibres, enable enhanced nonlinear optical effects and applications not currently possible with comparatively bulky optical fibres. Although microfibres have helped greatly to enhance the optical Kerr effect and stimulated Raman scattering for supercontinuum generation [18] , [19] , Brillouin scattering (BS) in these tiny waveguides has not been explored yet. Until now, only transverse acoustic resonances have been reported in long optical fibre tapers with a large diameter of a few micrometres [20] . In this work, we present what is to our knowledge the first complete measurement and numerical modelling of Brillouin scattering in a subwavelength-diameter optical fibre, revealing the full elastic wave distribution of such tiny optical waveguides. More specifically, we demonstrate the all-optical generation of a new class of surface acoustic waves (SAWs) and report the observation of SAW Brillouin scattering (SAWBS) in the backward direction. In addition to surface waves, our experimental and theoretical investigations also show that silica microwires also exhibit several widely spaced Brillouin frequencies involving hybrid shear and LAWs, as previously demonstrated in small-core PCFs [2] . Our experimental measurements are checked against numerical simulations of the equations of elastodynamics including the electrostrictive stress. Principle Let us first describe the opto-mechanical interaction under consideration. When coherent laser light is coupled and guided into a long uniform optical microwire as that shown schematically in Fig. 1 , the light both excites and feels several types of elastic waves with similar micrometre-scale wavelengths. In standard optical fibres, the light is guided into the core and is therefore solely sensitive to both shear and longitudinal bulk acoustic waves, leading to well-known physical effects such as guided acoustic wave Brillouin scattering [21] and stimulated Brillouin scattering [22] (SBS), respectively. In contrast, in subwavelength-diameter optical fibres, the guided light and particularly the evanescent field interact with the outer surface. Light can thus shake the wire and generate SAWs. The associated mechanical ripples will lead to small periodic changes of the effective refractive index along the optical microwire. When passing through this moving refractive index grating, light undergoes Bragg scattering in the backward direction according to the phase-matching condition, as in fibre-based Brillouin scattering from LAWs. The backscattered Brillouin signal also undergoes a slight shift of its carrier frequency due to the Doppler effect according to the photon–phonon energy conservation law ν B =2 n eff V / λ , with n eff , the effective refractive index of the microwire; λ , the optical wavelength in vacuum and V, the acoustic phase velocity. The acoustic velocity however significantly differs for surface, shear and longitudinal waves. Surface waves travel at a velocity between 0.87 and 0.95 of a shear wave (for fused silica, V S =3,400 m s −1 ). This gives rise to new optical sidebands down-shifted from 6 GHz in the light spectrum ( Fig. 1c ). On top of surface waves, there are also bulk hybrid acoustic waves (HAW) involving both shear and longitudinal components because of the mechanical boundary conditions [2] ( Fig. 1b ). HAWs propagate at an intermediate speed between shear and longitudinal waves with acoustic frequencies ~9 GHz. Furthermore, the sound energy density of surface waves is confined at the air–silica interface of the microwire, leading to small mechanical ripples of a few picometre, whereas, the HAW energy density remains trapped within the core without altering the wire shape ( Fig. 1c ). 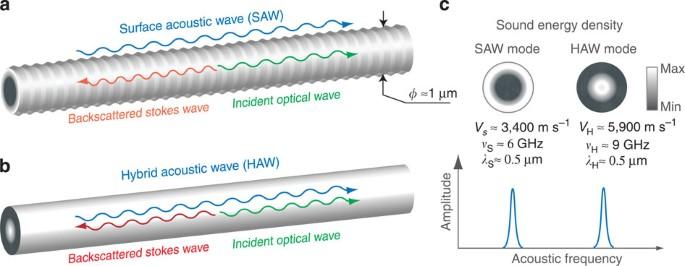Figure 1: Illustration of surface and hybrid acoustic wave Brillouin scattering in silica microwire. (a) Schematic representation of the silica microwire and of the wavevector interaction for surface acoustic waves (SAW). (b) Same for hybrid acoustic waves (HAW). (c) Comparison of sound energy densities, acoustic velocities and Brillouin frequency shifts between surface and hybrid waves. The surface wave is confined below the microwire surface and gives rise to small mechanical ripples, whereas the hybrid bulk wave remains confined within the core without altering the microwire surface. Figure 1: Illustration of surface and hybrid acoustic wave Brillouin scattering in silica microwire. ( a ) Schematic representation of the silica microwire and of the wavevector interaction for surface acoustic waves (SAW). ( b ) Same for hybrid acoustic waves (HAW). ( c ) Comparison of sound energy densities, acoustic velocities and Brillouin frequency shifts between surface and hybrid waves. The surface wave is confined below the microwire surface and gives rise to small mechanical ripples, whereas the hybrid bulk wave remains confined within the core without altering the microwire surface. Full size image Experimental setup In our experiment, we investigated several subwavelength-diameter silica optical fibres, as those shown schematically in Fig. 2a and in the image of Fig. 2c . They were drawn from a commercial single-mode fibre (SMF) using the heat-brush technique [23] , [24] (for details, see Fabrication method). They have a waist diameter ~1 μm, a length of 8 cm and the input/output tapered fibre sections are 15-mm long. 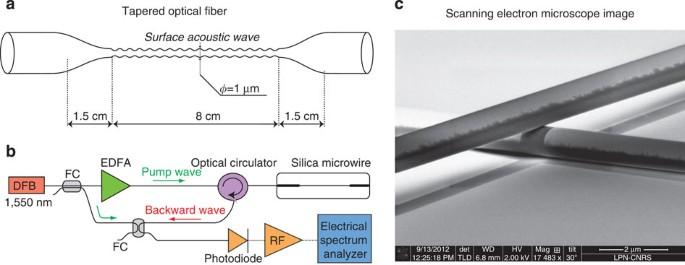Figure 2: Experimental implementation for backward Brillouin scattering detection in silica microwire. (a) Schematic of the tapered silica microwire. (b) Experimental setup. The backscattered light from the microwire is mixed with the input and the Brillouin signal is detected using a fast photodiode and an electrical spectrum analyser. DFB, distributed-feedback laser. FC, 10:90 fibre coupler. EDFA, Erbium-doped fibre amplifier. (c) Scanning electron microscope (SEM) image of typical silica wire. Courtesy of A.-L. Coutrot and C. Dupuis. Figure 2b shows the experimental setup to detect Brillouin backscattering [25] . As a pump laser, we used a narrow-linewidth continuous-wave distributed-feedback laser running at a wavelength of 1,550 nm. The laser output was split into two beams using a fibre coupler. One beam was amplified and injected in the optical microwire through an optical circulator, while the other beam served for detection. We then implemented a heterodyne detection in which the backscattered light from the microwire was mixed with the input coming from a second fibre coupler. The resulting beat note was then detected using a fast photodiode and averaged Brillouin spectra recorded using an electrical spectrum analyser. Figure 2: Experimental implementation for backward Brillouin scattering detection in silica microwire. ( a ) Schematic of the tapered silica microwire. ( b ) Experimental setup. The backscattered light from the microwire is mixed with the input and the Brillouin signal is detected using a fast photodiode and an electrical spectrum analyser. DFB, distributed-feedback laser. FC, 10:90 fibre coupler. EDFA, Erbium-doped fibre amplifier. ( c ) Scanning electron microscope (SEM) image of typical silica wire. Courtesy of A.-L. Coutrot and C. Dupuis. 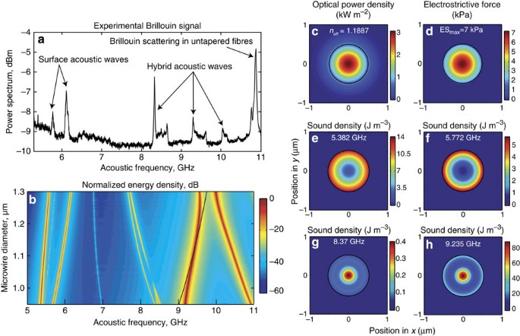Figure 3: Observation of Brillouin scattering in silica microwire. (a) Experimental Brillouin spectrum measured with a continuous-wave laser at 1,550 nm in a 8-cm long silica optical microwire with a diameter of 1 μm (See experimental setup for details). (b) Numerical simulations of Brillouin scattering spectrum for a microwire waist varying from 1 to 1.35 μm (See numerical method). The black line shows the acoustic frequency given by the phase-matching condition for pure longitudinal waves (kA=2kp). (c) Optical power density in the fundamental TE-like mode at a wavelength of 1,550 nm (neff=1.1887). (d) Spatial distribution of the electrostrictive stress under 1 W optical power. (e,f) Sound density of surface acoustic waves at 5.382 and 5.772 GHz. (g,h) Sound density of hybrid bulk acoustic modes at 8.37 and 9.235 GHz. Full size image Experimental results Figure 3a shows the experimental Brillouin spectrum for an input power of 100 mW and for a wire diameter of 1 μm. We see the clear emergence of several frequency peaks with different weights and linewidths in a radio-frequency range from 6 to 11 GHz. First, the high frequency at 10.86 GHz originates from standard Brillouin scattering in the 2-m-long untapered fibre sections and can be disregarded. More importantly, three other peaks appear at 8.33, 9.3 GHz, and slightly >10 GHz, respectively. The two first peaks exhibit a linewidth ~25 MHz, in good agreement with the acoustic amplitude lifetime in fused silica (~10 ns). On the basis of numerical simulations described below, we identified them as resulting from Brillouin scattering from hybrid waves whereas the two other resonances ~6 GHz are clearly the signature of SAWs. Figure 3: Observation of Brillouin scattering in silica microwire. ( a ) Experimental Brillouin spectrum measured with a continuous-wave laser at 1,550 nm in a 8-cm long silica optical microwire with a diameter of 1 μm (See experimental setup for details). ( b ) Numerical simulations of Brillouin scattering spectrum for a microwire waist varying from 1 to 1.35 μm (See numerical method). The black line shows the acoustic frequency given by the phase-matching condition for pure longitudinal waves ( k A =2 k p ). ( c ) Optical power density in the fundamental TE-like mode at a wavelength of 1,550 nm ( n eff =1.1887). ( d ) Spatial distribution of the electrostrictive stress under 1 W optical power. ( e , f ) Sound density of surface acoustic waves at 5.382 and 5.772 GHz. ( g , h ) Sound density of hybrid bulk acoustic modes at 8.37 and 9.235 GHz. Full size image Numerical simulations To better understand the nature of these acoustic modes, we performed numerical simulations on the basis of the equations of elastodynamics extended to account for electrostriction, a key physical effect in Brillouin scattering whereby matter become compressed under the effect of an electric field [26] , [27] (for details, see Numerical method section). With respect to standard three-wave mixing SBS theory [28] , this new modelling provides an excellent estimate of the theoretical Brillouin gain spectrum by computing the energy density of acoustic phonons generated by light. We considered the silica microwire as a rod-type cylinder and we took into account all elastic and optical parameters of silica. For the sake of simplicity, we neglected the two conical tapered sections of the fibre taper. We must also stress that we did not include in our model the radiation pressure induced by light at the surface of the microwire due to Maxwell stress. Using the method described in ref. 29 , we have indeed theoretically estimated that the radiation pressure is <1% of the electrostrictive stress in silica wire of 1 μm diameter. Radiation pressure should, however, be taken into account for nanowires whose diameter is <500 nm. The results of our numerical simulations are shown in Fig. 3b–h . The elastic energy is plotted in Fig. 3b versus acoustic frequency and for a wire diameter varying from 1 to 1.35 μm. As can be seen, we retrieve most of the surface and hybrid acoustic resonances, as those observed experimentally in Fig. 3a . There are, however, slight differences with experiment regarding the precise acoustic resonant frequencies. We attribute them to both the microwire uniformity and diameter uncertainty. Nevertheless, we can clearly identify two surface acoustic modes ~6 GHz, and three hybrid acoustic modes ~9 GHz. More information is provided by the modal distribution of the interacting waves. Figure 3c shows the spatial distribution of the optical mode intensity in the waist region at a wavelength of 1,550 nm. The black circle marks out the interface between silica and air. The optical mode is guided in the microwire with a rather long evanescent tail extending outside silica. The tight confinement of the optical field into the microwire induces an electrostrictive stress ~30 times larger than in usual optical fibre (up to 7 kPa as compared with 250 Pa under same incident optical power [26] ). As a comparison, the radiation pressure is only 50 Pa at the surface of microwire. The electrostrictive stress distribution, shown in Fig. 3d , follows the optical mode distribution without extending out of the microwire. The sound energy density of the two SAWs at 5.382 GHz and 5.772 GHz are plotted in Fig. 3e,f for a waist of 1.05 μm. As can be seen, the elastic energy density is mainly localized below the wire surface. In contrast, the kinetic energy density of HAWs at 8.37 and 9.235 GHz, shown in Fig. 3g,h , are mostly confined within the core of the taper. The role of confining elastic energy is due to the elastic waveguide properties of such microwires, mostly its small diameter and hard mechanical boundary conditions. To go further into details, we plot in Fig. 4a the full elastic wave spectrum over a wider range of wire diameter till 3.6 μm. For every diameter, the fundamental optical mode is recomputed and normalized. The refractive index n eff increases smoothly with the diameter as the optical mode becomes more and more localized within silica rather than air. The two SAWs that we identified before exist for every diameter with a slight shift in frequency. Their acoustic energy is significant for small core but strongly reduces as the diameter increases beyond the optical wavelength (1.5 μm). This observation is consistent with the simultaneous decrease of the overlap of SAW with the fundamental optical mode guided inside the core. 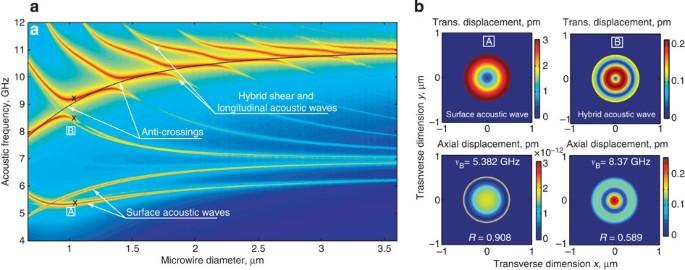Figure 4: Numerical simulations of the full acoustic wave spectrum and displacements in silica microwire. (a) Colour plot of energy density of acoustic waves as a function of frequency and for a wire diameter varying from 0.6 to 3.5 μm. The black curve shows the acoustic frequency given by the standard phase-matching condition (kA=2kp) for pure longitudinal waves. White arrows indicate the surface and hybrid acoustic waves, and the anti-crossing points due to the strong coupling regime. (b) Transverse (trans.) and axial displacements in the microwire associated with surface and hybrid acoustic modes labelled A and B ina. Figure 4a also shows that, for a given microwire diameter, multiple HAW with widely spaced frequencies can be simultaneously excited, as in small-core PCFs [2] , [5] . This means that, in such small subwavelength waveguides, the light–sound interaction is fundamentally different from standard optical fibres. Brillouin spectrum is not simply the signature of a single bulk longitudinal sound wave. In such tiny waveguides, instead, waveguide boundary conditions induce a strong coupling of shear and longitudinal displacements, resulting in a much richer dynamics of light interaction with hybrid and SAWs. We can thus see the emergence of several avoided crossings and acoustic resonance splitting in Fig. 4a , due to the fact that HAWs are not orthogonal and thus strongly interact. This interaction is strong enough for certain acoustic frequencies to be forbidden at some anti-crossing points, as shown by the white arrows in Fig. 4a . In contrast, the two SAW branches cross without interacting for a diameter ~0.85 μm because they have orthogonal polarizations. Figure 4b shows the associated transverse and axial displacements in the microwire for one of surface and hybrid modes, denoted A and B in Fig. 4a . Transverse and axial displacements are simply defined as and (| u z |), respectively. R is defined as the ratio between spatial integrals of the shear and longitudinal displacements ( R =1 for a pure shear wave). As can be seen, the surface acoustic mode A at 5.382 GHz exhibits a transversal displacement of a few picometres and a weak axial displacement just below the wire surface. Clearly, this is the signature of a surface Rayleigh wave that combines both a longitudinal and transverse motion to create mechanical ripples with an elliptic orbit motion. In contrast, the displacements for the hybrid mode B are smaller ( R =0.589) and mainly localized within the core of the wire. Figure 4: Numerical simulations of the full acoustic wave spectrum and displacements in silica microwire. ( a ) Colour plot of energy density of acoustic waves as a function of frequency and for a wire diameter varying from 0.6 to 3.5 μm. The black curve shows the acoustic frequency given by the standard phase-matching condition ( k A =2 k p ) for pure longitudinal waves. White arrows indicate the surface and hybrid acoustic waves, and the anti-crossing points due to the strong coupling regime. ( b ) Transverse (trans.) and axial displacements in the microwire associated with surface and hybrid acoustic modes labelled A and B in a . Full size image One may then wonder what is the scattering efficiency and if the threshold for stimulated regime is raised for SAWBS. To answer these important issues, we have estimated the Brillouin gain from the experimental spectrum in Fig. 3a . Starting from the usual theory of Brillouin scattering [30] , the Brillouin gain g B can be expressed as , where n eff is the effective refractive index of the microwire, P 12 is the elasto-optic constant and ρ is the mean density of fused silica (SiO 2 ), c is the speed of light in vacuum, λ is the optical wavelength, ν B and Δ ν B are the SAW frequency shift and FWHM width of the spectrum. From measurements, we get ν B =5.85 GHz and Δ ν B =20 MHz for the first SAW peak, thus we found g B =1.4.10 −12 m W −1 , to be compared with g B =3.10 −11 m W −1 for SMF fibres. If we now consider the effective mode area A eff to get the Brillouin gain factor by unit length, we found that g B / A eff =8 W −1 m −1 for a 1-μm-diameter silica wire whereas it is only 0.4 W −1 m −1 for SMF fibres. That clearly means that the scattering efficiency is rather high. When examining carefully the spectrum of Fig. 3a , one can indeed clearly see that the SAW efficiency in the microwire is just 2-dB below that of Brillouin scattering in the 2 m-long fibre pigtails. However the threshold for stimulated regime is not raised over so short propagation distance. It can readily be derived from the Brillouin gain using the following standard formula [30] P th =(21 A eff )/( Kg B L eff ), where L eff is the effective length that accounts for losses and K the polarization factor ( K =1.5). Assuming 10 dB of linear losses for the microwire from measurements, we found a high threshold power of P th =60 W in silica microwire which is well above the continuous-wave power used in the experiment (100 mW). This high threshold power level could, however, be achieved using amplified long nanosecond optical pulses instead of continuous-wave power. There also could be improvement in microwire parameters such as optical loss. In addition, we can expect that the surface Brillouin threshold can be substantially reduced in optical microwire made of highly nonlinear chalcogenide glasses [10] , [31] . In conclusion, we have reported a clear-cut evidence of a new type of Brillouin light scattering driven by SAWs by use of a subwavelength-diameter silica fibre. It has been further shown that the SAWs reported here travel the wire surface at a specific velocity of 3,400 m s −1 and give rise to new useful optical sidebands around 6 GHz in the scattering spectrum. This work thus may represent a landmark to foster the investigation of such surface waves in many different photonic platforms, such as PCFs and integrated optical devices (for example, chalcogenide and silicon chips). In addition, SAWBS can find strong potential applications for optical sensing and detection because these acoustic waves are inherently sensitive to surface features and defects and are already used in many sensing systems (for example, MEMS). They could be seen as a new class of Brillouin optical sensors that rely on the modulation of SAWs to sense a physical phenomenon (for example, temperature, stress, gas). Changes in amplitude and frequency of the Brillouin signal through the silica microwire could be advantageously used to measure the presence of the desired phenomenon. One can also imagine a strong interaction between surface waves and surface plasmons by depositing a thin layer of gold or silver [32] , [33] . These results thus show the potential of optical microwires and nanowires for surface Brillouin scattering [34] , optical sensing and nonlinear plasmonics [32] , [33] . Finally, this work contributes to the further understanding of the intriguing light–sound interactions in subwavelength optics and in nanophotonics. Fabrication method The silica microwire has been tapered from a standard telecom fibre (SMF-28) using the heat-brush technique [24] . The fibre to be pulled is attached at two computer-controlled translation stages. The fibre is softened on its central part with a small butane flame. The gas flow is monitored and regulated by a mass-flow controller. The flame is kept fixed while the two translation stages elongate the fibre to create the microwire. The microwire shape is fully controlled by the trajectories of the two translation stages. The untapered parts, upstream and downstream the microwire, allow a very easy light injection and collection. During the pulling, a laser light is coupled inside the microwire and collected at the output end to control several parameters (transmitted power, mode shape and spectrum). With this home-made pulling platform, we routinely achieved light transmission larger than 90% over the full fibre including the tapered and untapered parts, even with microwire diameters of a few hundred nanometres and lengths up to several centimeters. Numerical method Our experimental observations of surface and HAWs are modelled with the equations of elastodynamics including the electrostrictive stress induced by the optical field. Specifically, the displacements u i in silica microwire are given by a simple partial differential equation which reads: where c ijkl is the rank-4 tensor of elastic constants. is the eletrostrictive stress tensor, with the rank-4 susceptibility tensor χ klij = ε km ε ln p mnij and p mnij the elasto-optic tensor. ε 0 is the permitivity of vacuum. The force term with detuning frequency ω = ω 1 − ω 2 is proportional to with k = k 1 − k 2 . Here we assume that the total optical field results from the superposition of the pump and Brillouin Stokes waves with angular frequencies ω 1,2 and axial wavevectors k 1,2 . If the two optical waves are propagating in opposite directions (See Fig. 1a,b ) k ≈2 k 1 and we speak of backward SBS or SAWBS. We also consider in our model the phonon lifetime by taking into account the elastic losses assuming a complex tensor. This loss model is compatible with the usual assumption that the product of the quality factor Q and the acoustic frequency is a constant for a given material (for example, for silica, Q × f=5 THz). Further applying Green’s theorem to equation (1), we get which accounts for the theorem of virtual work for the elestrostrictive stress. For numerical computations, we used the Galerkin nodal finite element method to transform the integral equation into the following linear matrix system with mass matrix M , stiffness matrix K ( k )= K 0 + kK 1 + k 2 K 2 , and X ( k )= X 0 + kX 1 . U is the vector norm of nodal displacements ū i . Solutions of equation (3) as a function of frequency detuning yield rigorous distribution of displacements within microwire cross-section as shown in Fig. 3 . The associated sound energy density can be directly compared with experimental measurements of Brillouin scattering. Finally, the electrostriction stress tensor is defined by the optical modal distribution ( Fig. 3c,d ), which is beforehand calculated using a finite element method (Comsol software). How to cite this article: Beugnot, J.-C. B. et al. Brillouin light scattering from surface acoustic waves in a subwavelength-diameter optical fibre. Nat. Commun. 5:5242 doi: 10.1038/ncomms6242 (2014).